The emergence of modern sea ice cover in the Arctic Ocean Arctic sea ice coverage is shrinking in response to global climate change and summer ice-free conditions in the Arctic Ocean are predicted by the end of the century. The validity of this prediction could potentially be tested through the reconstruction of the climate of the Pliocene epoch (5.33–2.58 million years ago), an analogue of a future warmer Earth. Here we show that, in the Eurasian sector of the Arctic Ocean, ice-free conditions prevailed in the early Pliocene until sea ice expanded from the central Arctic Ocean for the first time ca. 4 million years ago. Amplified by a rise in topography in several regions of the Arctic and enhanced freshening of the Arctic Ocean, sea ice expanded progressively in response to positive ice-albedo feedback mechanisms. Sea ice reached its modern winter maximum extension for the first time during the culmination of the Northern Hemisphere glaciation, ca. 2.6 million years ago. Quantitative determination of past sea ice coverage in the Arctic Ocean is critically important for future climate predictions, as sea ice constrains the effect of changing surface albedo, ocean–atmosphere heat exchanges and potential freshwater export to the North Atlantic which, in turn, influences the meridional overturning circulation (MOC) and thus, global climate [1] . Through the Integrated Ocean Drilling Program Arctic Coring Expedition [2] , the prevalence of sea ice in the central Arctic Ocean since the middle Miocene (~18 Ma) has been established previously [3] , [4] , [5] , although new research proposes the ephemeral presence of perennial sea ice as early as 36 Ma (ref. 6 ). A reduction in sea ice cover has been reported during the upper Miocene [7] and the Pliocene [8] , and modelling experiments indicate that the removal of Arctic sea ice around the early-to-late Pliocene transition (~3.6 Ma) explains the proxy-based high paleotemperature reconstruction in the Canadian high Arctic [9] , [10] . Other simulations, however, reveal reduced, but still significant Arctic sea ice cover during the same period [11] . Dowsett et al . [12] concluded that the present discrepancy between Pliocene sea surface temperature (SST) proxy estimates and model simulations in the high latitudes requires a further refinement of the current model parameterization. Since Pliocene sequences in the Arctic are incomplete, the spatial and temporal evolution of SST and sea ice extent remains, however, largely uncertain. In the current study, we investigated long-term changes in Arctic sea ice coverage at its present summer ice margin in the Atlantic—Arctic gateway (AAG) region using borehole data that expose a complete marine Pliocene sequence. Ocean Drilling Program Hole 910C (80°15.896 ′N, 6°35.430 ′E, 556 m water depth) and Hole 911 A (80°28.466 ′N, 8°13.640 ′E, 902 m water depth) were recovered from the eastern flank of the Yermak Plateau, NW Spitsbergen ( Fig. 1 ) [13] . This region is particularly well suited for the study of sea ice limits in the Arctic Ocean because it is located within the spatial and temporal dynamics of the inflow of warm Atlantic water and outflow of cold Arctic water masses via the Transpolar Drift ( Fig. 1 ). In recent years, the analysis of the biomarker IP 25 (‘Ice Proxy with 25 carbon atoms’) [14] , a mono-unsaturated highly branched isoprenoid lipid biosynthesized by certain sea ice diatoms [15] , has become an established proxy method for the reconstruction of Arctic sea ice [16] . The presence (absence) of IP 25 in Arctic marine sediments is especially sensitive to the past occurrence (absence) of sea ice [16] , while abundance variations are usually consistent with corresponding directional changes in sea ice cover [16] . These attributes are of particular significance to the current study, as it has previously been shown that ice marginal conditions in the gateway (Fram Strait) are mirrored, qualitatively, by the occurrence of IP 25 in marine sediments from the study region, and that sedimentary abundances of IP 25 are sensitive to changes in sea ice conditions [17] , [18] , thus permitting semi-quantitative reconstructions. As a result, the measurement of IP 25 in AAG sediments covering the last 2 Ma has been used to imply marginal sea ice conditions during the Pleistocene [19] . The new IP 25 record from the AAG shows that sea ice expanded from the Arctic Ocean to its modern limits for the first time ca. 4 million years ago. We suggest that a rise in topography above a critical threshold for ice accumulation in several regions of the Arctic, together with enhanced freshwater delivery to the Arctic Ocean during the early Pliocene preconditioned the northern landmasses to become recipients for glacial ice during the late Pliocene. To complement the IP 25 record, we also studied the distributions of glycerol dialkyl glycerol tetraethers (GDGTs) and hydroxyl GDGTs to infer changes in SST [20] . 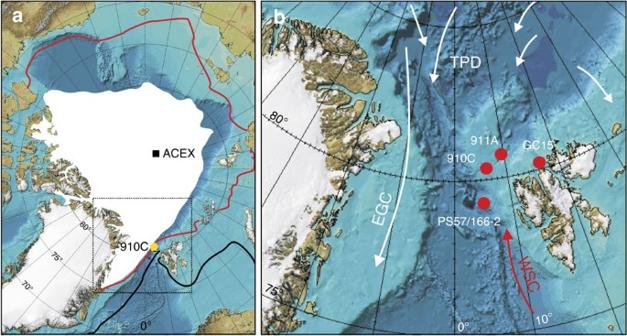Figure 1: Physiogeography of the Arctic Ocean. (a) Bathymetry and modern sea ice limit (white polygon) in September 2012 (National Snow and Ice Data Center (NSIDC)). Minimum (red line) and maximum (black line) sea ice extent for the interval 1981–2010 are also indicated (NSIDC). Locations of Ocean Drilling Program (ODP) Hole 910C and Integrated ODP Expedition 302 (ACEX—Arctic Coring Expedition) are indicated. (b) Surface currents in the Atlantic-Arctic gateway (TPD, Transpolar Drift; EGC, East Greenland Current; WSC, West Spitsbergen Current) and surface samples from two locations (PS57/166-2, 79°13 ′N, 4°89′E; GC15, 80°51′N, 15°9′E with IP25concentrations of 0.0086 and 0.0117 μg g−1sed., respectively. Locations of ODP Leg 151 Hole 910C and 911A are displayed. Figure 1: Physiogeography of the Arctic Ocean. ( a ) Bathymetry and modern sea ice limit (white polygon) in September 2012 (National Snow and Ice Data Center (NSIDC)). Minimum (red line) and maximum (black line) sea ice extent for the interval 1981–2010 are also indicated (NSIDC). Locations of Ocean Drilling Program (ODP) Hole 910C and Integrated ODP Expedition 302 (ACEX—Arctic Coring Expedition) are indicated. ( b ) Surface currents in the Atlantic-Arctic gateway (TPD, Transpolar Drift; EGC, East Greenland Current; WSC, West Spitsbergen Current) and surface samples from two locations (PS57/166-2, 79°13 ′N, 4°89′E; GC15, 80°51′N, 15°9′E with IP 25 concentrations of 0.0086 and 0.0117 μg g −1 sed., respectively. Locations of ODP Leg 151 Hole 910C and 911A are displayed. Full size image Borehole chronology The chronostratigraphic framework in Hole 910C indicates the recovery of a complete Pliocene sequence [21] with the age model revealing a consistently high sedimentation rate (6–16 cm per kyr) [22] . The age model is based on new paleomagnetic and biostratigraphic data of Hole 910C and nearby Hole 911A ( Fig. 1 ), and correlated into high-resolution seismic data across the Yermak Plateau [22] ( Supplementary Table 1 ). 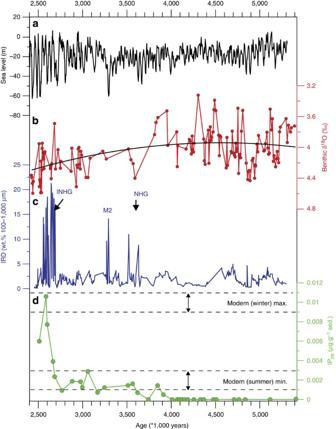Figure 2: Pliocene proxy data from the AAG. (a) Pliocene sea level record29derived from global marine isotope stack23. (b) Stable oxygen isotopes (δ18O) of benthic foraminiferaCassidulina teretisin Ocean Drilling Program (ODP) Hole 910C. Black line indicates the second-degree polynomial function. (c) Ice-rafted debris (IRD; wt.%, coarse fraction 100–1,000 μm) recorded from the eastern AAG (ODP Hole 911A; ref.21). Black arrows indicate the intensification of the Northern Hemisphere Glaciation (INHG) at ~2.64 Ma (ref.25), as well as the onset of the Northern Hemisphere Glaciation (NHG) sensu Mudelsee and Raymo27. Marine Isotope Stage M2 glaciation at ~3.30 Ma is also displayed. (d) IP25concentrations in ODP Hole 910C. Values representing proposed summer and winter sea ice limits in the study region are indicated by stippled lines. Additional fix points were derived from correlating the global marine stack of δ 18 O records [23] with new benthic δ 18 O data of Hole 910C ( Supplementary Table 2 ). The benthic δ 18 O isotope record shows a gradual trend from lower (~3.5–4.0‰) to higher (~4.0–4.5‰) values from the early to the late Pliocene ( Fig. 2 ), supporting the changes observed elsewhere in the Nordic Seas, with similar or significantly less ice volume occurring during the early Pliocene compared with the late Pliocene [24] . The cooling in the late Pliocene can also be inferred from the record of ice-rafted debris (IRD; Fig. 2 ), which shows the largest IRD pulses concomitant with the intensification of the Northern Hemisphere Glaciation (INHG) at ~2.64 Ma (ref. 25 ), and occasional smaller IRD pulses at ~3.3 Ma (marine isotope stage M2 glaciation) [26] and ~3.6 Ma (onset of Northern Hemisphere Glaciation (NHG) sensu Mudelsee and Raymo [27] ). The latter is consistent with a distinct change from lower (3.6‰) to higher δ 18 O values (4.4‰) and falling sea level (−20 m; refs 28 , 29 ; Fig. 2 ), thus supporting inferences of enhanced ice volume in the Northern Hemisphere since ~3.6 Ma (refs 27 , 30 ). Figure 2: Pliocene proxy data from the AAG. ( a ) Pliocene sea level record [29] derived from global marine isotope stack [23] . ( b ) Stable oxygen isotopes (δ 18 O) of benthic foraminifera Cassidulina teretis in Ocean Drilling Program (ODP) Hole 910C. Black line indicates the second-degree polynomial function. ( c ) Ice-rafted debris (IRD; wt.%, coarse fraction 100–1,000 μm) recorded from the eastern AAG (ODP Hole 911A; ref. 21 ). Black arrows indicate the intensification of the Northern Hemisphere Glaciation (INHG) at ~2.64 Ma (ref. 25 ), as well as the onset of the Northern Hemisphere Glaciation (NHG) sensu Mudelsee and Raymo [27] . Marine Isotope Stage M2 glaciation at ~3.30 Ma is also displayed. ( d ) IP 25 concentrations in ODP Hole 910C. Values representing proposed summer and winter sea ice limits in the study region are indicated by stippled lines. Full size image Pliocene sea ice record for the Arctic Ocean Our IP 25 sea ice reconstruction for the Fram Strait indicates ice-free conditions at the borehole location between 5.8 and 3.9 Ma, as inferred from the absence of IP 25 ( Figs 2 and 3 ). This contrasts with the modern setting, where IP 25 has been detected in surface sediments from the region consistent with the site being located between the winter and summer sea ice limits ( Fig. 1 ) [18] . The failure to detect IP 25 in sediments between 5.8 and 3.9 Ma may, potentially, also be explained by the occurrence of perennial sea ice coverage. However, this is unlikely since the interval is near the warm period around the early/late Pliocene transition (~3.6 Ma) recorded in the high Arctic [10] , with mean annual temperatures significantly warmer than present [10] , [31] . The occurrence of the phytoplanktic sterol brassicasterol (a proxy indicator of open-water conditions [18] ) ( Fig. 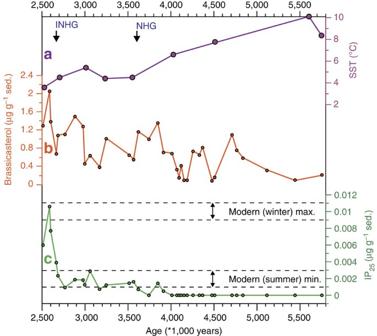Figure 3: Surface water conditions in the AAG during the Pliocene. (a) Sea surface temperature (SST) estimates. Values are based on distributions of GDGTs and hydroxyl GDGTs in Ocean Drilling Program (ODP) Hole 910C sediments (see Methods section for more details). Black arrows indicate the intensification of the Northern Hemisphere Glaciation (INHG) at ~2.64 Ma (ref.25), as well as the onset of the NHG sensu Mudelsee and Raymo27. (b) Brassicasterol (open-water indicator) concentrations. (c) IP25concentrations. Values representing proposed summer and winter sea ice limits in the study region are indicated by stippled lines. 3 and Supplementary Table 3 ) and elevated SST estimates based on distributions of GDGTs and hydroxyl GDGTs [32] , [33] ( Fig. 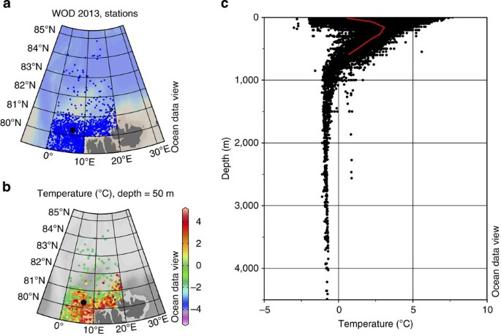Figure 4: Modern Oceanography. (a) Available stations in the study region stored in World Ocean Database (WOD) 2013. (b) Sea surface temperature (depth=50 m) distribution in the study region. Black circle indicates the position of ODP Hole 910C. (c) Temperature-Depth profile of all stations in the study region. Red line indicates the reference station at the borehole location (WOD13_DE) measured at 19 June 1984. 3 and Supplementary Table 4 ) also suggests an absence of perennial sea ice during the studied interval. Distributions of the hydroxyl GDGTs, in particular, indicate relatively warm conditions (ca. 7–10 °C and Fig. 3 ), implying a dominance of Atlantic water rather than polar water during the early Pliocene in the AAG region. Figure 3: Surface water conditions in the AAG during the Pliocene. ( a ) Sea surface temperature (SST) estimates. Values are based on distributions of GDGTs and hydroxyl GDGTs in Ocean Drilling Program (ODP) Hole 910C sediments (see Methods section for more details). Black arrows indicate the intensification of the Northern Hemisphere Glaciation (INHG) at ~2.64 Ma (ref. 25 ), as well as the onset of the NHG sensu Mudelsee and Raymo [27] . ( b ) Brassicasterol (open-water indicator) concentrations. ( c ) IP 25 concentrations. Values representing proposed summer and winter sea ice limits in the study region are indicated by stippled lines. Full size image The first occurrence of IP 25 at ca. 3.9 Ma provides clear evidence for the emergence of seasonal sea ice at the borehole location, and thus a gradual expansion of Arctic sea ice cover ( Fig. 2 ). Following this onset, IP 25 concentrations remain relatively low between ca. 3.9 and 3.0 Ma, consistent with less sea ice coverage during the warm periods around the early/late Pliocene transition and the mid-Piacenzian warm period from 3.29 to 2.97 Ma (refs 10 , 30 , 34 , 35 ) with sea ice conditions probably similar to the modern (summer) minimum ( Fig. 1 ). Nevertheless, there is a gradual increase in IP 25 concentration up to ca. 2.7 Ma, before a more rapid increase to modern maximum (winter) levels (ca. 0.01 μg g −1 sed.) ( Fig. 2 ) [18] found in nearby surface sediments ( Fig. 1 ), suggesting a phased expansion towards contemporary sea ice conditions at ca. 2.6 Ma, coincident with the INHG (that is, glaciation to mid-latitudes) at ca. 2.64 Ma (ref. 25 ). A semi-quantitative assessment of past sea ice conditions in the AAG expressed by the PIP 25 index [18] suggests an extensive sea ice cover after ~2.68 Ma as indicated by PIP 25 values >0.7 ( Supplementary Fig. 1 ). IP 25 concentrations are also similar to modern values over the last 2 Ma on the Yermak Plateau [19] , and the new IP 25 record suggests the establishment of the modern sea ice limits ( Fig. 1 ) at ca. 2.6 Ma. Further, SST estimates based on hydroxyl GDGTs (ca. 3.5–5.5 °C; Fig. 3 and Supplementary Table 4 ) fall within the range of modern summer SSTs on the southern Yermak Plateau ( Fig. 4 ), indicating substantial cooling and increasing influence of polar water masses parallel to the onset of the NHG at ~3.6 Ma. Coldest SSTs (~3.5 °C) after the INHG ( Fig. 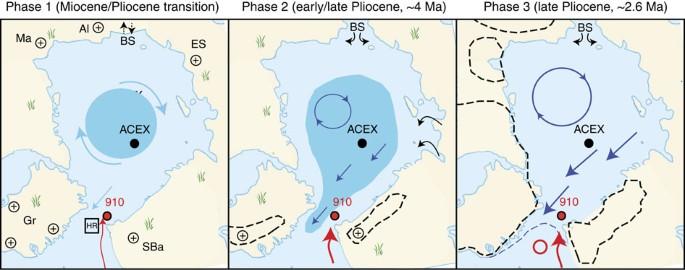Figure 5: Development of modern sea ice cover during the Pliocene. (Phase 1) Perennial sea ice in the Arctic interior during the Miocene/Pliocene transition. Late Miocene/early Pliocene tectonic uplift in circum-Arctic (crosses) is recorded in the Svalbard/Barents Sea region (SBa), on Greenland (Gr), Mackenzie Region (Ma), Alaska (Al) and East Siberia (ES)21,44,47,48. Early Pliocene vegetation is characterized by taiga forests with dominantPiceaandPinus36. Restricted deep/shallow water exchange through Atlantic-Arctic gateway (HR, Hovgaard Ridge)21and Bering Strait (BS)38,39,40,41. (Phase 2) Arctic sea ice expanded to its modern summer limits for the first time after ~4 Ma. Pre-glacial uplift reached a threshold for ice-growth (stippled lines). Enhanced thermohaline circulation (red/blue arrows in AAG)46,51and freshening of the Arctic through BS and Siberian rivers51,57(black arrows). (Phase 3) Expansion of Arctic sea ice to its modern winter limits at ~2.6 Ma. Stippled blue line indicates the modern winter sea ice limits in the AAG. Large-scale ice sheets recorded in Eurasia21, Greenland54and North America70close to potential moisture sources in the Nordic seas (red open circle)54and subarctic Pacific Ocean56. Limits of glacial ice extent are relative and do not show their actual size. 3 ) approach contemporary GDGT–SST estimates observed in nearby surface sediments ( Supplementary Table 5 ). Figure 4: Modern Oceanography. ( a ) Available stations in the study region stored in World Ocean Database (WOD) 2013. ( b ) Sea surface temperature (depth=50 m) distribution in the study region. Black circle indicates the position of ODP Hole 910C. ( c ) Temperature-Depth profile of all stations in the study region. Red line indicates the reference station at the borehole location (WOD13_DE) measured at 19 June 1984. Full size image The implications of these observations are threefold: phase 1 (M/P boundary) is characterized by a dense vegetation cover in the high northern latitudes, predominantly taiga forests with dominant Picea and Pinus [36] , and a reduction of the Greenland Ice Sheet by at least 30% (ref. 37 ). At this time, the Arctic Ocean was partly isolated, with restricted AAG through-flow [21] , and the Bering Strait still in the initial opening phase [38] , [39] , [40] , [41] . The prevalence of an estuarine circulation in the Arctic Ocean [42] , [43] , together with a high continental mean annual temperature (MAT) would have restricted the occurrence of sea ice in the Arctic interior. As such, the marginal seas (including the study location here) would have been ice-free or covered by first-year winter sea ice only ( Fig. 5 ). Figure 5: Development of modern sea ice cover during the Pliocene. (Phase 1) Perennial sea ice in the Arctic interior during the Miocene/Pliocene transition. Late Miocene/early Pliocene tectonic uplift in circum-Arctic (crosses) is recorded in the Svalbard/Barents Sea region (SBa), on Greenland (Gr), Mackenzie Region (Ma), Alaska (Al) and East Siberia (ES) [21] , [44] , [47] , [48] . Early Pliocene vegetation is characterized by taiga forests with dominant Picea and Pinus [36] . Restricted deep/shallow water exchange through Atlantic-Arctic gateway (HR, Hovgaard Ridge) [21] and Bering Strait (BS) [38] , [39] , [40] , [41] . (Phase 2) Arctic sea ice expanded to its modern summer limits for the first time after ~4 Ma. Pre-glacial uplift reached a threshold for ice-growth (stippled lines). Enhanced thermohaline circulation (red/blue arrows in AAG) [46] , [51] and freshening of the Arctic through BS and Siberian rivers [51] , [57] (black arrows). (Phase 3) Expansion of Arctic sea ice to its modern winter limits at ~2.6 Ma. Stippled blue line indicates the modern winter sea ice limits in the AAG. Large-scale ice sheets recorded in Eurasia [21] , Greenland [54] and North America [70] close to potential moisture sources in the Nordic seas (red open circle) [54] and subarctic Pacific Ocean [56] . Limits of glacial ice extent are relative and do not show their actual size. Full size image During phase 2 (early/late Pliocene transition), changing tectonic boundary conditions in the circum-Arctic during the late Miocene-early Pliocene, including mountainous uplift [44] and open/closing gateways (AAG, Bering Strait, Central American Seaways (CAS)) [21] , [45] , [46] , triggered the expansion of the Arctic sea ice coverage, reaching the modern summer limit ( Fig. 1 ) for the first time at ca. 3.9 Ma ( Fig. 5 ). This timing is consistent with recent inferences on tectonic uplift events on Greenland [47] , the Barents Sea [21] and Arctic Canada [48] , when elevated plateaus became available to host perennial ice fields and, ultimately, continental ice. The expansion of sea ice in the Arctic at this time parallels the increased low-saline Arctic through-flow via Bering Strait as documented by a major invasion of Pacific mollusks to the North Atlantic from ~4.4 to 4.5 Ma (ref. 49 ). The evidence of an oscillating West Antarctic ice sheet [50] and sea level variations on average by ±20 m around the modern level until 3.3 Ma (refs 28 , 29 ; Fig. 2 ) suggest that, between 5.0 and 3.9 Ma, the Bering Strait was mostly submerged. Enhanced freshwater delivery to the Arctic via Siberian rivers associated with the advancing closure of the CAS and increased MOC between 4.7 and 4.5 Ma (refs 46 , 51 , 52 ) further facilitated sea ice formation in the Arctic Ocean and supports the inferred establishment of the ‘modern-type’ East Greenland Current between 4.5 and 4.3 Ma (ref. 21 ). The enhanced sea ice export through the (now) established deep-water AAG counterbalanced the heat transport associated with the enhanced MOC owing to the closure of the CAS. In contrast, modern sea ice limits, with the margin located above the borehole location throughout most of the year, were not reached until the INHG at ca. 2.64 Ma (phase 3) ( Fig. 5 ). The unprecedented long period of ice marginal conditions in the AAG parallel to the INHG confirms the amplification of polar cooling in response to internal feedbacks superimposed on the long-term decrease in atmospheric CO 2 concentration and slow tectonic forcings [27] , [53] . Among the array of feedbacks that are debated, the most sensitive for sea ice and glacial ice conditions in the AAG region are likely changes in the MOC in response to the final closure of the CAS after ca. 2.9 Ma (ref. 54 ). That the closure and associated enhanced MOC is unable to produce large-scale ice sheets in numerical models [55] may be owing to the use of similar to modern boundary conditions (gateways and orography) for the Pliocene. However, adjusting the models for orographic changes over Greenland, and the exposed landmasses of northern Eurasia above a threshold for glacial ice accumulation and massive winter sea ice coverage since ca. 4 Ma ( Fig. 5 ), may allow models to simulate enhanced MOC and more precipitation over Greenland and reproduce the formation of large-scale ice sheets. The additional effect of the irreversible closure of the CAS after ca. 2.9 Ma (that is, increased poleward atmospheric moisture transport—both in the AAG and the subarctic Pacific [56] ) induced a freshening of the Arctic Ocean [54] , as evidenced by the rapid spatial and temporal expansion of its sea ice cover. These, in turn, strengthened the sea ice export via the East Greenland Current, promoted ice-albedo feedback mechanisms and thermally isolated Greenland; thus, fostering build-up of continental ice sheets in the circum-Arctic during the INHG. The pre-requisite for these marked changes in the polar ocean-ice-continent climate system, however, were orographic changes in the circum-Arctic and freshening of the Arctic Ocean during the early Pliocene. Pre-glacial uplift and final deepening of the gateways preconditioned the landmasses to become recipient for glacial ice. Before the closure of the CAS as an additional amplifier for Arctic freshening and sea ice expansion [57] , we suggest that tectonic forcing in the Arctic was the decisive factor responsible for climate deterioration in the Northern Hemisphere. Finally, the new sea ice reconstruction for the Pliocene Arctic Ocean provides a new dimension for paleoclimate modelling to reproduce a warm climate state in Earth history such as the mid Pliocene warmth [34] . Thus, by demonstrating that sea ice in the Eurasian sector of the Arctic existed along its modern summer limit during the most recent interval of long-term average warmth relative to the last million years, climate simulations, with fully proxy-consistent boundary conditions for the Arctic Ocean, can be further refined to improve validation of projected climate for the end of the current century [1] . Stable isotope analyses The new stable isotope data set of the benthic foraminifera Cassidulina teretis test (100–1,000 μm fraction) was generated at the Leibniz Laboratory for Radiometric Dating and Stable Isotope Research in Kiel, Germany, using a Finnigan MAT 251 isotope ratio gas mass spectrometer, directly coupled to an automated carbonate preparation device (Kiel I prototype) and calibrated using NIST19 international standard to the Vienna Peedee belemnite scale. The precision of the measurements at 1σ based on repeated analyses of internal laboratory standards was better than ±0.07‰ and ±0.05‰ for oxygen and carbon isotopes, respectively. Because C. teretis secretes its carbonate close to oxygen isotopic equilibrium with the ambient seawater, no further corrections or adjustments were applied to the δ 18 O data [58] . Biomarker analyses IP 25 was extracted, identified and quantified according to the methods of Belt et al . [59] with minor modifications. Briefly, 9-octylheptadec-8-ene (10 μl; 10 μg ml −1 ) was added as an internal standard to each freeze-dried sediment sample (2–3 g) to permit subsequent quantification by gas chromatography—mass spectrometry (GC–MS). Sediments were then extracted using a mixture of dichloromethane/methanol (2:1, v/v) and ultrasonication (15 min), and the resulting solutions were decanted and dried (N 2 ) to yield a total organic extract (TOE). Before analysis of TOEs using GC–MS, it was necessary to first remove elemental sulphur that was present in relatively high concentrations in the majority of the extracts. This was achieved by first re-dissolving the TOEs in hexane (1 ml) and adding tetrabutylammonium sulphite (1 ml) and 2-propanol (2 ml). The resulting suspensions were then agitated by hand (1 min) before addition of a further 3 ml of water and re-agitated (1 min). Samples were then centrifuged (2 min) and the surface (hexane) layer containing IP 25 was transferred to a clean vial. The aqueous phase was extracted twice more (hexane; 2 × 1 ml). Following removal of hexane from the combined extracts (nitrogen; room temperature), nonpolar lipids (including IP 25 ) were obtained using open-column chromatography (silica; 6 ml hexane). These partially purified nonpolar lipid fractions were further separated into saturated and unsaturated hydrocarbons using glass pipettes containing silver ion solid phase extraction material (Supelco discovery Ag-ion). Saturated hydrocarbons (hexane; 5 ml, then dichloromethane; 5 ml) and unsaturated hydrocarbons including IP 25 (dichloromethane/acetone (95/5); 10 ml) were eluted as consecutive fractions. Individual hydrocarbon fractions were analysed by GC–MS with operating conditions as described previously, for example, ref. 59 . Mass spectrometric analysis was carried out in total ion current and single-ion monitoring (SIM) modes. IP 25 was identified on the basis of its characteristic GC retention index and mass spectrum obtained from a laboratory standard ( Supplementary Fig. 2 ). The identification of IP 25 was further confirmed by hydrogenation (PtO 2 .2H 2 O; H 2 ; 30 min) to the parent C 25 highly branched isoprenoid alkane, which was identified on the basis of its own characteristic retention index and mass spectrum and by comparison of each of these with those obtained from a laboratory standard. Quantification was achieved by dividing the integrated GC–MS peak area of IP 25 by that of the internal standard (9-octylheptadec-8-ene; both m/z (mass to charge ratio) 350) and normalizing this ratio using an instrumental response factor obtained from laboratory standards of each analyte [59] and the mass of sediment. The analytical reproducibility (7%, n =3) was determined using a standard sediment with a known concentration of IP 25 . The limit of detection ( s / n =3) for IP 25 was 0.5 ng g −1 dry sediment based on extraction of 2 g sediment and concentration of partially purified sediment extracts to 20 μl before analysis by GC–MS. Analysis of brassicasterol was carried out as per Belt et al . [60] Calculation of PIP 25 values was performed according to Müller et al . [18] For the GDGTs analyses, freeze-dried sediment samples (3–6.7 g) were extracted with a solvent mixture of dichloromethane/methanol (3:1,v/v) using microwave assisted extraction in a MARS X System (CEM, Matthews, NC, USA). After centrifugation and evaporation of the solvent, the extracts were separated into four fractions using 1% deactivated SiO 2 column chromatography. The eluents were hexane, hexane/dichloromethane (2:1, v/v), dichloromethane and dichloromethane/methanol (95:5, v/v). GDGTs were obtained in the fourth fraction, dried under gentle N 2 -stream, re-dissolved in hexane/n-propanol (99:1, v/v) and filtered through 0.50 μm polytetrafluoroethylene (PTFE) filters (Advantec). Extracts were then eluted through a Tracer Excel CN column (0.4 × 20 cm, 3 μm; Teknokroma), equipped with a pre-column filter and a guard column using high-performance liquid chromatography coupled to mass spectrometry (HPLC-MS). using an atmospheric pressure chemical interphase. The solvent programme was adapted from Schouten et al . [61] and Escala et al . [62] Samples were eluted with hexane/n-propanol at 0.6 ml min −1 . The amount of n -propanol was held at 1.5% for 4 min, increased gradually to 5.0% during 11 min, then increased to 10% during 1 min and held at 10% for 4 min, then decreased to 1.5% during 1 min and held at 1.5% for 9 min until the end of the run. The parameters of the atmospheric pressure chemical interphase were set as follows to generate positive ion spectra: corona discharge 3 μA, vaporizer temperature 400 °C, sheath gas pressure 49 mTorr, auxiliary gas (N 2 ) pressure 5 mTorr and capillary temperature 200 °C. Isoprenoid GDGTs were monitored in selected ion monitoring (SIM) mode at m/z 1,302, 1,300, 1,298, 1,296 and 1,292. The hydroxyl GDGTs were monitored in SIM mode at m/z 1,318 and 1,316. The identification of the hydroxyl GDGTs at m/z 1,318 and 1,316 has been described in Huguet et al . [33] The HPLC–MS system was checked for TEX 86 index accuracy with a standard sediment sample before and between sample sets [63] . The synthetic tetraether lipid GR was used as external standard. Compound GR has an m/z of 1,208, a structure typical of neutral archaeal membrane lipids and presumably does not occur in the environment [63] , [64] . External curves were measured before each sample series. The reproducibility of the quantification is estimated to be ±10%. When temperatures are expected to fall below 15 °C, Kim et al . [65] recommended the use of the TEX 86 L index to estimate past SST (error estimates (1 sigma) are given as 4 °C (ref. 65 )): TEX 86 L =log[GDGT2/(GDGT1+GDGT2+GDGT3)]; SST=67.5 × TEX 86 L +46.9 ( r 2 =0.86, n =396, P <0.0001). It should be noted, however, that SST estimates derived from both TEX 86 or TEX 86 L may be anomalously high in the Arctic, especially in the vicinity of Siberian river mouths and the sea ice margin [66] . A modified TEX 86 index and calibration (TEX 86 ′) had been proposed and applied for Arctic Ocean (~87.5° N) temperatures during the Palaeocene/Eocene thermal maximum [67] : TEX 86 ′=[(GDGT2+GDGT3+Cren′)/(GDGT1+GDGT2+Cren′)]; TEX 86 ′=0.016 × SST+0.20 ( R 2 =0.93). TEX 86 ′, however, also yields anomalously high temperatures in Hole 910C ( Supplementary Table 4 ). The recently discovered hydroxyl GDGTs [68] have been shown to infer SSTs on a global scale [33] and to indicate the presence of polar waters in the Arctic Ocean [32] . Fietz et al . [32] proposed a so-called OH-GDGT% index and a promising SST calibration (slightly modified from Huguet et al . [33] ) based on the hydroxyl and isoprenoid GDGTs: OH-GDGT%=(Σ hydroxyl GDGTs)/(Σ hydroxyl GDGTs+Σ isoprenoid GDGTs); OH-GDGT%=8.6–0.67 × SST ( R 2 =0.55, P =0.004, n =11). The OH-GDGT% index yields reasonable SSTs for Hole 910C ( Supplementary Tables 4 and 5 ) even though absolute values must be confirmed in larger surface sediment data sets. Modern oceanography Modern SST (depth=50m) data from the study region were extracted from the World Ocean Database (WOD 2013) and displayed by ODV version 4.6.2 (ref. 69 ). How to cite this article: Knies, J. et al . The emergence of modern sea ice cover in the Arctic Ocean. Nat. Commun. 5:5608 doi: 10.1038/ncomms6608 (2014).